3D multifunctional integumentary membranes for spatiotemporal cardiac measurements and stimulation across the entire epicardium Means for high-density multiparametric physiological mapping and stimulation are critically important in both basic and clinical cardiology. Current conformal electronic systems are essentially 2D sheets, which cannot cover the full epicardial surface or maintain reliable contact for chronic use without sutures or adhesives. Here we create 3D elastic membranes shaped precisely to match the epicardium of the heart via the use of 3D printing, as a platform for deformable arrays of multifunctional sensors, electronic and optoelectronic components. Such integumentary devices completely envelop the heart, in a form-fitting manner, and possess inherent elasticity, providing a mechanically stable biotic/abiotic interface during normal cardiac cycles. Component examples range from actuators for electrical, thermal and optical stimulation, to sensors for pH, temperature and mechanical strain. The semiconductor materials include silicon, gallium arsenide and gallium nitride, co-integrated with metals, metal oxides and polymers, to provide these and other operational capabilities. Ex vivo physiological experiments demonstrate various functions and methodological possibilities for cardiac research and therapy. Tools for cardiac physiological mapping are indispensable for the clinical identification and mechanistic understanding of excitation–contraction coupling, metabolic dysfunction, arrhythmia and other conditions. Devices developed in the 1980s attempted to address this need by using synthetic fabrics sewn to loosely resemble the shape of the ventricle, with bulk electrodes manually assembled and woven into this platform [1] , [2] , [3] , [4] . Although such schemes provide some utility, they do not enable uniform quality of contact across the heart high-density mapping capabilities, provision for multifunctional recordings, precision measurement/stimulation or practical deployment as chronic implants. As a result, alternative strategies based on serial mapping with point-contact catheters or on imaging techniques that use fluorescence, nuclear magnetic resonance or ultrasound have emerged, even though each has significant shortcomings [5] , [6] , [7] , [8] . The ideal scenario remains one in which device functionality integrates directly and non-invasively with the heart, suitable for chronic use. The essential challenge is that the heart is a complex electromechanical syncytium with numerous elements working in synchrony to reliably pump blood and respond to changing metabolic demands. Although much has been gained from isolated cellular studies, the integral functional behaviour on the organ level and the interaction between the electrical, metabolic and mechanical remodelling in disease states, especially in vivo , remain poorly explored due to paucity of adequate tools. Thus, there is an unmet need for multiparametric mapping capabilities inclusive but far beyond electrical sensing in a conformal, high-resolution manner, which cannot be realized using conventional materials, device technologies or imaging modalities. Recent developments in materials and mechanics concepts for stretchable electronics [9] , [10] , [11] , [12] , [13] , [14] create an opportunity to meet this challenge of direct, full three-dimensional (3D) integration of devices with the epicardial surface. Here we expand on previously reported small-scale electronic devices as two-dimensional (2D) flexible sheets [15] , to build multifunctional semiconductor systems in lithographically defined configurations on 3D, thin elastic membranes, custom-formed to match the shape of the heart. The physical format resembles that of the naturally occurring membrane that surrounds the heart, known as the pericardium. These systems, which we refer to as 3D multifunctional integumentary membranes (3D-MIMs) provide conformal interfaces to all points on the heart, with robust but non-invasive contacts enabled by the soft elasticity of the membrane itself, throughout dynamic cardiac cycles, even when completely immersed in fluid media. Measurements on isolated perfused rabbit hearts demonstrate the utility of these ideas as a general platform for multifunctional, high-density epicardial mapping/stimulation. The results provide advanced methodological possibilities for basic and clinical cardiology. Design and fabrication The fabrication begins with the creation of a thin, 3D elastic membrane shaped to the heart. As shown in Fig. 1a , optical segmentation techniques first capture the full 3D geometry of a heart of interest [16] . A commercial 3D printer (ZPrinter 450, Z-Corporation) then renders a solid model of the heart in a proportionally scaled form, as described later, to serve as a substrate for mounting ultrathin electronic/optoelectronic and sensor systems, separately prefabricated on planar substrates. Casting and curing a thin layer of silicone elastomer on top of the heart model with these multifunctional devices on its surface defines the overall format. The front faces of the device components contact the model while the back faces bond to the elastomer. Removing the system (that is, 3D membrane with integrated device components) from the model prepares it for installation around a living heart, as a type of ‘instrumented’, artificial pericardium. 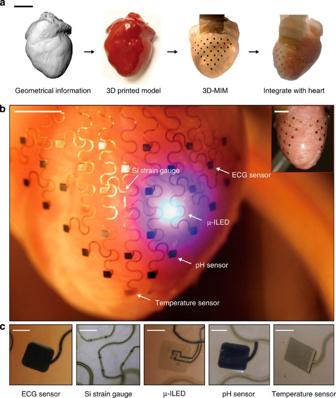Figure 1: 3D-MIMs for spatiotemporal measurement and stimulation across the entire epicardial surface. (a) Graphical depiction of the key steps in device design and fabrication. Scale bar, 2 cm. (b) Images of a representative 3D multifunctional integumentary membrane (3D-MIM) integrated on a Langendorff-perfused rabbit heart. The white arrows highlight various function elements in this system. The electronics can cover both anterior and posterior surfaces of the heart (inset). Scale bars, 6 mm. (c) Magnified views of the functional elements in conformal contact with the epicardium. The images are recorded from the back side of the devices. Scale bars, 500 μm. Figure 1: 3D-MIMs for spatiotemporal measurement and stimulation across the entire epicardial surface. ( a ) Graphical depiction of the key steps in device design and fabrication. Scale bar, 2 cm. ( b ) Images of a representative 3D multifunctional integumentary membrane (3D-MIM) integrated on a Langendorff-perfused rabbit heart. The white arrows highlight various function elements in this system. The electronics can cover both anterior and posterior surfaces of the heart (inset). Scale bars, 6 mm. ( c ) Magnified views of the functional elements in conformal contact with the epicardium. The images are recorded from the back side of the devices. Scale bars, 500 μm. Full size image Figure 1b shows a representative 3D-MIM that includes microscale, inorganic light-emitting diodes (μ-ILEDs) based on indium gallium nitride (InGaN) for optical mapping, silicon (Si) nanomembranes for strain gauges, gold (Au) electrodes for electrical sensing/stimulation, iridium oxide (IrO x ) pads for pH sensors and Au serpentine resistors for temperature sensors/heaters. The methods for creating these components exploit modern integrated circuit technologies and achieve spatial resolution far beyond that possible with manually assembled arrays. A thin, flexible heat-seal conductive cable (Elform, HST-9805-210) serves as a connection to external hardware for data acquisition, power supply and control. The 3D-MIM is engineered with overall dimensions slightly smaller than those of the real heart, to provide adequate elasticity and mechanical support for robust contact with the epicardium during diastole and systole, but with sufficiently small pressures to avoid disruption of natural behaviours of the cardiac tissue. The serpentine mesh that interconnects the device components covers the ventricle and conforms to the contours of the epicardium. Although this example is designed for research applications on rabbit hearts, the same strategies are applicable to human hearts, or even other organ systems. Here the 3D geometries can be obtained using similar 3D-printed substrates with patient-specific MRI or CT organ segmentation. Mechanical analysis A critical feature of this type of device is that it can be designed to maintain a stable mechanical interface to the tissue while exerting minimal force on the contracting and relaxing heart muscle. In the cardiac anatomy of humans and other vertebrates, the myocardium is enclosed in a space sealed by the pericardium, which allows reversible volume change within a certain range. When a pathophysiological condition leads to inflammation, the pericardium exerts pressure to constrain the motions of the heart chambers. Quantitative analysis allows a comparative assessment of the pressure associated with our 3D device membrane on the epicardium, as well as the dependence of this pressure on material properties and design parameters. 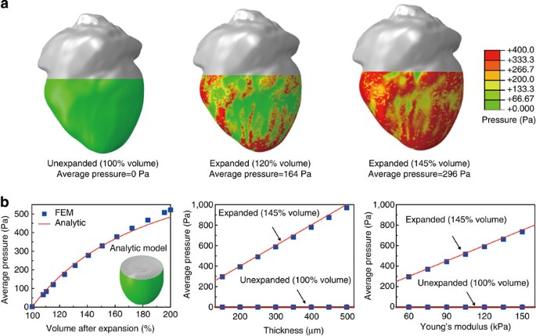Figure 2: Analysis of pressures on the epicardium associated with integration of a 3D-MIM. (a) Calculated pressure distribution induced by a device with total thickness of 150 μm and effective Young’s modulus of 60 kPa under various conditions of volume expansion of a heart geometry. (b) FEM and analytical results of average pressure as functions of volume expansion (left), thickness (middle) and Young’s modulus (right) of the membrane. Figure 2a shows results for a 3D-MIM with a membrane thickness of 150 μm and effective Young’s modulus of ~60 kPa (Ecoflex, Smooth-on) at various states of volume expansion (1+ ε ) 3 of a heart geometry, calculated using 3D finite element methods (FEM), where ε is the linear expansion factor. The thickness of the membrane is uniform in the analysis; the nonuniformity due to the electronic devices results in local increase of the effective Young’s modulus to ~80 kPa and adds <50% of the approximate pressure, as discussed in details in Methods section and Supplementary Fig. 1 . The form of the undeformed membrane follows that of a 3D model, proportionally size-reduced (~30% volume reduction compared with the diastolic state of the real heart) to ensure a baseline level of pressure upon application on the real heart. Computations correspond to the heart at its contracted volume (3D model), and at systolic (120% of the contracted volume) and diastolic (145% of the contracted volume) conditions. The calculated average pressures are similar to those of pericardium under normal physiological conditions, and only ~20% of these pressures are under conditions of pericardial constraint [17] , [18] , [19] , [20] , [21] , [22] . The results suggest that the device is unlikely to cause restrictive impact, as confirmed by ex vivo studies described subsequently. FEM and analytic modelling also establish general relationships between the pressure and the design parameters. Figure 2b shows the average pressure as a function of the volume expansion, the thickness of the membrane and its Young’s modulus. The analytic model uses a partial ellipsoid to approximate the geometry of the heart. Details appear in Methods section and Supplementary Fig. 1 . The following expression connects the average pressure, the membrane geometry, mechanical properties and expansion factor: Figure 2: Analysis of pressures on the epicardium associated with integration of a 3D-MIM. ( a ) Calculated pressure distribution induced by a device with total thickness of 150 μm and effective Young’s modulus of 60 kPa under various conditions of volume expansion of a heart geometry. ( b ) FEM and analytical results of average pressure as functions of volume expansion (left), thickness (middle) and Young’s modulus (right) of the membrane. Full size image where t is the thickness of the membrane, E and ν are the effective Young’s modulus and the Poisson’s ratio, respectively. The constant C decreases as the heart size increases, and C also depends on the shape of the heart (~0.2 mm −1 for a rabbit heart). Decreases in membrane thicknesses and Young’s moduli both linearly reduce the pressure. This scaling allows designs that provide pressures sufficiently large to maintain good contact between the sensor/actuator network and the epicardial surface, but sufficiently small to avoid impact on the intrinsic physiology. Monitoring the time course of several electrophysiological parameters that indicate ischaemia in an isolated pressure-loaded, working rabbit heart model [23] with and without a 3D-MIM reveals the effects. The results, based on control ( N =3) and experimental ( N =3) hearts ( Supplementary Fig. 2 ), suggest that there is no additional ischaemia caused by the devices, as measured by ST elevation and the amplitude of the LV pressure waveform. Spatiotemporal cardiac measurements and stimulation To demonstrate the various functional modes of operation we begin with high-precision mapping of epicardial electrical activity. These experiments, and all of those that follow, used explanted Langendorff-perfused rabbit hearts. The 3D geometrical information was obtained from a representative rabbit heart. A single 3D-MIM can accommodate some range in specific sizes and shapes associated with a single type of animal model, due to its soft, elastic construction. The device here incorporates 68 Au electrodes (1 mm 2 surface area and spacing of 3.5 mm), distributed across both the anterior and posterior surfaces of the epicardium ( Fig. 3a,d and Supplementary Fig. 3 ). The electrochemical impedances of individual electrodes are ~2 kΩ at a frequency of 1 kHz, measured in phosphate-buffered saline ( Supplementary Fig. 4 ). The transparency of the membrane allows simultaneous optical mapping through voltage-dependent fluorescence, as a means for validating the electrical measurements [5] . Experiments involved signals acquired from four hearts for a variety of conditions: normal sinus rhythms, and paced at a range of frequencies and from a range of electrode pairs to increase the variability of the propagation patterns in the spatial activation maps. The surface electrograms (EGs) captured various key morphologies associated with the QRS and T waves ( Fig. 3a ). Representative maps and correlations between electrical and optical activation times appear in Fig. 3c,b , respectively. The overall linear correlations between optical and electrical activation times were 0.957 for sinus data and 0.943 for paced data. These studies indicate that this configuration of measurement electrodes can replicate patterns of activation to a resolution that captures the spatial variations observed optically. Analyses for additional electrophysiological parameters are summarized in Supplementary Fig. 6 . 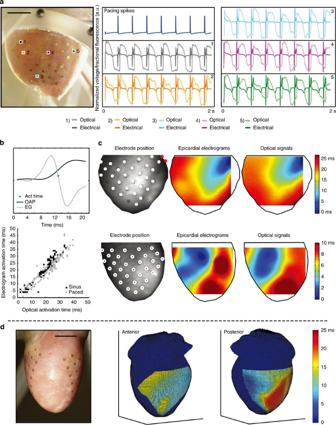Figure 3: High-density electrical mapping. (a) Representative optical and electrical signals acquired simultaneously from the corresponding numbered electrode locations on a Langendorff-perfused rabbit heart. Scale bar, 7 mm. (b) Top: schematic illustration of a representative optical action potential, unipolar EG and position of the activation time, defined asfor the optical action potential andfor the EG. Bottom: correlation of electrical and optical activation times for hearts tested in a variety of states. (c) Interpolated spatial activation maps determined from the electrical and optical measurements. Top: heart paced by the red pair of electrodes on the membrane. Bottom: sinus rhythm. (d) 3D mapping of electrical signalling from both the anterior and posterior surfaces of the heart. Interpolated spatial maps of electrical activation time are projected on a representative rabbit heart geometry, for purposes of visualization. Scale bar, 7 mm. Figure 3d presents a 3D map derived from signals recorded from the anterior and posterior surfaces of the heart. Unlike optical mapping where motion artefacts dramatically impact the measurement quality requiring static heart geometries, electrophysiological mapping with 3D-MIMs can be applied under normal beating condition. As shown in Supplementary Video , the integrated sensors move synchronously with the underlying cardiac tissue. Although it is practically difficult to avoid relative lateral motion between the sensors and the epicardium during beating cycles, due to the engineered geometries of 3D-MIMs, the displacement can be minimized to be less than the characteristic sizes of the sensors and to have negligible impact to the signal quality ( Supplementary Fig. 5 ). This feature is necessary for extending the mapping capabilities beyond laboratory studies and implementing in clinical electrophysiology. Figure 3: High-density electrical mapping. ( a ) Representative optical and electrical signals acquired simultaneously from the corresponding numbered electrode locations on a Langendorff-perfused rabbit heart. Scale bar, 7 mm. ( b ) Top: schematic illustration of a representative optical action potential, unipolar EG and position of the activation time, defined as for the optical action potential and for the EG. Bottom: correlation of electrical and optical activation times for hearts tested in a variety of states. ( c ) Interpolated spatial activation maps determined from the electrical and optical measurements. Top: heart paced by the red pair of electrodes on the membrane. Bottom: sinus rhythm. ( d ) 3D mapping of electrical signalling from both the anterior and posterior surfaces of the heart. Interpolated spatial maps of electrical activation time are projected on a representative rabbit heart geometry, for purposes of visualization. Scale bar, 7 mm. Full size image Mapping of changes in pH provides useful information on the metabolic state of the heart. Here iridium oxide (IrO x ), a well-established material for pH sensing, enables the measurement [24] . Electrodeposited IrO x on Au electrodes provides pH sensors with average open circuit potential responses of 68.9 mV per pH with s.d. of 8.6 mV per pH for 32 sensors over the array at 37 °C in Tyrode’s solution ( Supplementary Fig. 7 ). The temperature dependence of the pH sensors is nearly −1.6±0.02 mV °C −1 (μ± σ ), which corresponds to ~0.02 pH for a 1 °C change in temperature. Temperature variations over a physiologically relevant range will, therefore, have a small effect on the pH measurement. For cases where large changes in temperature are externally introduced, the temperature dependence of the pH sensor must be accounted for explicitly. Such pH sensors, along with optical mapping techniques, enable acquisition of maps of pH, transmembrane potential ( V m ) and calcium transient (CaT) signals during global no-flow ischaemia–reperfusion. The pH sensors cover the left anterior and posterior surface of the rabbit heart ( Fig. 4a ). At baseline, all pH sensors record values between 7.34 and 7.40. The responses of two pH sensors (highlighted by grey and charcoal colours) are plotted ( Fig. 4b ) throughout the protocol. Complete spatial pH maps at time points t 1 (baseline), t 2 (10 min into ischaemia) and t 3 (20 min into reperfusion) appear in Fig. 4d–f (left). Turning off the perfusion pump immediately reduced coronary pressure to 0 mm Hg and led to an approximately linear decrease in pH to minimum values of 6.40 (grey) and 6.22 (charcoal). Upon reperfusion, the pH rapidly increased until initiation of ventricular tachycardia where the pH stabilized at levels somewhat below baseline values. A sample far-field ECG of reperfusion-induced ventricular tachycardia appears in Fig. 4c . After spontaneous conversion back to sinus rhythm, the pH values increased again to pre-ischemic values. 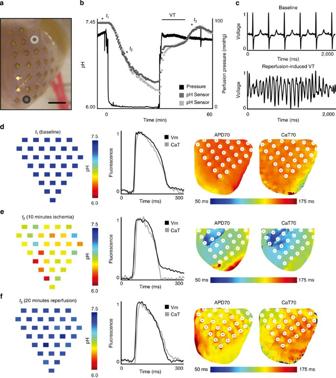Figure 4: High-density pH and optical mapping of transmembrane potential and calcium transients. (a) 3D-MIM with pH sensors array integrated on a Langendorff-perfused rabbit heart with 2 pH sensors highlighted and values displayed in (b). Scale bar, 7 mm. (b) Temporal change in pH during 30 min of no-flow ischaemia followed by 30 min of reperfusion. Three times starred ast1,t2andt3correspond to spatial pH maps in (d–f). (c) Representative far-field ECG during baseline and reperfusion-induced ventricular tachycardia (VT). (d–f) pH map of 32 sensors (left), representative transmembrane potential and calcium transient signals (middle), and APD70–CaT70 maps (right) at baseline (d), 10 min of no-flow ischaemia (e) and 20 min of reperfusion (f). The results provide maps of the anterior–posterior LV. TheVmand CaT are taken from the same pixel, but the location may vary slightly due to shrinkage of the heart during no-flow ischaemia. White circles denote pH sensors positions. VT, ventricular tachycardia;Vm, transmembrane potential; CaT, calcium transient; APD70, action potential duration at 70% repolarization; CaT70, calcium transient duration at 70% relaxation. Figure 4d–f shows pH maps (left), representative optical signals ( V m —black and CaT—grey; middle) and side-by-side action potential duration at 70% repolarization (APD70) and calcium transient duration at 70% return to baseline (CaT70) maps. At the baseline, pH, APD70 and CaT70 maps highlight that the pH and electrophysiological parameters were initially uniform over the surface of the heart. After 10 min of ischaemia, pH, APD70 and CaT70 changed, though not in a spatially uniform manner. CaT alternans (short and long duration) were observed during ischaemia and here we show a short CaT70 in Fig. 4e . After 20 min of reperfusion, parameters returned to values close to the baseline levels. This experiment demonstrates possibilities in multiparametric mapping during ischaemia/reperfusion. The information establishes anatomical relationships between metabolism and excitation–contraction coupling. Figure 4: High-density pH and optical mapping of transmembrane potential and calcium transients. ( a ) 3D-MIM with pH sensors array integrated on a Langendorff-perfused rabbit heart with 2 pH sensors highlighted and values displayed in ( b ). Scale bar, 7 mm. ( b ) Temporal change in pH during 30 min of no-flow ischaemia followed by 30 min of reperfusion. Three times starred as t 1 , t 2 and t 3 correspond to spatial pH maps in ( d – f ). ( c ) Representative far-field ECG during baseline and reperfusion-induced ventricular tachycardia (VT). ( d – f ) pH map of 32 sensors (left), representative transmembrane potential and calcium transient signals (middle), and APD70–CaT70 maps (right) at baseline ( d ), 10 min of no-flow ischaemia ( e ) and 20 min of reperfusion ( f ). The results provide maps of the anterior–posterior LV. The V m and CaT are taken from the same pixel, but the location may vary slightly due to shrinkage of the heart during no-flow ischaemia. White circles denote pH sensors positions. VT, ventricular tachycardia; V m , transmembrane potential; CaT, calcium transient; APD70, action potential duration at 70% repolarization; CaT70, calcium transient duration at 70% relaxation. Full size image A 3D-MIM with arrays of temperature sensors illustrates capabilities in monitoring spatial distributions of cardiac temperature. The temperature sensor elements use designs established previously, consisting of serpentine traces of gold (20 μm wide, 50 nm thick) ( Supplementary Fig. 8 ) in which changes in resistance correlate to changes in temperature [25] . The temperature sensors exhibit linear responses over physiological range, with a measurement precision of ~23 mK when sampled at 2 Hz in typical hospital settings. 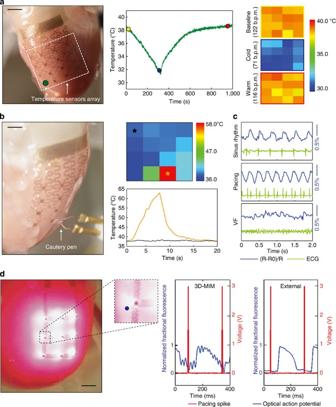Figure 5: Temperature and strain sensing combined with imaging enabled by integrated μ-ILEDs. (a) Application of a 3D-MIM for temperature monitoring during cold perfusion. Left: image of a 3D-MIM with 4 × 4 temperature sensors array integrated on a Langendorff-perfused rabbit heart. Middle: temperature recordings from a representative sensor illustrated in the left inset. Right: temperature maps at representative time points in the middle inset with corresponding heart rate calculated from ECG. Each pixel in the colour map corresponds to recording from one temperature sensor. Scale bar, 1 cm. (b) Temperature measurements during an ablation experiment. Positions of the sensor array and cautery pen are shown in the left inset. Temperature map during ablation (upper right) and recordings from representative sensors (bottom right) are shown respectively. Scale bar, 7 mm. (c) Responses of a Si strain sensor under representative physiological conditions, compared with simultaneous ECG recordings. (d) Left: image of a 3D-MIM with μ-ILEDs array in optical mapping experiments. Inset shows a magnified view of area around a representative μ-ILED. Right: comparison of optical signals from a representative pixel (blue dot on the left inset) recorded during excitation using μ-ILEDs on 3D-MIM and external optical excitation, respectively. Scale bar, 3 mm. Figure 5a shows a 3D-MIM with 16 integrated temperature sensors during use on a beating heart. The sensors are calibrated in temperature-controlled water bath before the animal experiments, exhibiting average responses of 1.23 Ω °C −1 with s.d. of 0.05 Ω °C −1 over 16 sensors across the array ( Supplementary Fig. 9 ). In one experiment, the temperature of the heart was changed by altering the temperature of the perfusion. As shown in Fig. 5a , the measured epicardial temperature gradually decreased by ~7°C during cooling of the perfusate, with a uniform distribution of temperature across the heart. The heart rate, determined from the far-field EG, decreased with decreasing temperature and recovered to the original value as the temperature returned to physiological levels, indicating that temperature controlled the rate of myocardial metabolism. In a second experiment, a cautery pen was used to acutely burn a small region of the epicardium, simulating clinical ablation. The associated temperature map ( Fig. 5b ) shows localized elevation of temperature near the point of ablation. Such information can be used as feedback for clinical control of ablation time and size of affected area. In combination with electrical sensors, such a device could provide the real-time relation between temperature and excitation. Figure 5: Temperature and strain sensing combined with imaging enabled by integrated μ-ILEDs. ( a ) Application of a 3D-MIM for temperature monitoring during cold perfusion. Left: image of a 3D-MIM with 4 × 4 temperature sensors array integrated on a Langendorff-perfused rabbit heart. Middle: temperature recordings from a representative sensor illustrated in the left inset. Right: temperature maps at representative time points in the middle inset with corresponding heart rate calculated from ECG. Each pixel in the colour map corresponds to recording from one temperature sensor. Scale bar, 1 cm. ( b ) Temperature measurements during an ablation experiment. Positions of the sensor array and cautery pen are shown in the left inset. Temperature map during ablation (upper right) and recordings from representative sensors (bottom right) are shown respectively. Scale bar, 7 mm. ( c ) Responses of a Si strain sensor under representative physiological conditions, compared with simultaneous ECG recordings. ( d ) Left: image of a 3D-MIM with μ-ILEDs array in optical mapping experiments. Inset shows a magnified view of area around a representative μ-ILED. Right: comparison of optical signals from a representative pixel (blue dot on the left inset) recorded during excitation using μ-ILEDs on 3D-MIM and external optical excitation, respectively. Scale bar, 3 mm. Full size image In addition to electrical and chemical evaluation, mechanical characteristics can be determined. Here strain sensors based on piezoresistive effects in nanomembranes of Si allow monitoring of the mechanics of contractions of the heart during a variety of propagation states. Careful mechanical design of the serpentine interconnect structures allows accurate measurement in spite of the fact that typical epicardial strains [26] greatly exceed the fracture threshold of Si, as described in previously reported small-scale 2D devices [15] . In the present design, the 3D-MIM strain sensors include three p-doped Si piezoresistors in a rosette configuration ( Supplementary Fig. 10 ). Two of the piezoresistors, with longitudinal axes perpendicular to each other, are aligned to the 110 crystalline directions of the Si, offering an effective longitudinal gauge factor of ~0.33 and effective transverse gauge factor of nearly −0.06 for each piezoresistor ( Supplementary Fig. 11 ). The piezoresistor aligned to the 100 crystalline direction exhibits relatively small change in resistance under strain, due to the intrinsic sensitivity associated with the crystalline direction as well as the overall device geometry. The piezoresistors aligned to the 110 directions provide maximum sensitivity for characterization of mechanical rhythms of the heart while the piezoresistor aligned to the 100 direction can be used to calibrate for effects of temperature. Experiments revealed the mechanical behaviours during sinus rhythm, ventricular pacing and pharmacologically induced ventricular fibrillation (VF) with Pinacidil (30 μM bulk dose). The use of Pinacidil significantly reduces the action potential duration and subsequently increases the vulnerability to reentrant arrhythmias when stimulated with 50 Hz A/C burst pacing. Bath electrodes simultaneously recorded a far-field ECG to establish the temporal correlation between the electrical and mechanical behaviour. Figure 5c shows the response of a representative piezoresistor aligned to the 110 direction. The measurements reveal mechanical rhythms of the cardiac cycles, with consistent cycling with ECG recordings. During VF condition, both the strain gauges and ECG show that the waveform lost normal rhythm and displayed a random pattern typical for VF. A final demonstration exploits arrays of μ-ILEDs [27] , [28] to illustrate the capacity for advanced semiconductor integration and optical mapping/stimulation. Here nine ultrathin (3 μm), microscale (300 × 300 μm 2 ) LEDs based on aluminium indium gallium phosphide (AlInGaP) with peak emission wavelengths of 670 nm ( Supplementary Figs 12 and 13 ) served as local light sources for the excitation of voltage-sensitive dyes. Changes in fluorescence associated with these dyes allowed measurement of the cardiac action potential. Figure 5d compares signals obtained with an external light source (Prizmatix, 630 nm) and with the integrated μ-ILEDs. In spite of their small sizes, the LEDs enable recording of clear action potentials, with waveform shapes consistent with external light. The signal-to-noise ratio of the μ-ILED-excited action potentials is lower than the externally excited action potentials due to a necessary decrease in light intensity to minimize the power delivered to the device. The results demonstrate the future possibility of an in vivo optical mapping using either externally applied dyes or internal fluorescent indicators and/or stimulation system in a 3D integration format. The results presented here suggest routes for integrating active electronic materials and sensors in 3D, organ-specific designs, with potential utility in both biomedical research and clinical applications. With attention to materials, engineering mechanics and functional devices, these systems can establish conformal interfaces with the epicardium, and perform a variety of high-density physiological multiparametric mapping and stimulation. The use of transfer printing and the reported scheme for integration onto the printed 3D heart structure allows diverse sensor/actuator devices on a single platform. Separate electrical connection, with a single trigger channel to synchronize the timing, eliminates effects of crosstalk. The devices can provide local information on the metabolic, excitable, ionic, contractile and thermal state for investigations of both the spatial and temporal responses to a variety of insults, diseases and therapies. The devices could be used to identify critical regions that indicate the origin of pathophysiological conditions such as arrhythmias, ischaemia or heart failure. These regions could then be used to guide therapeutic interventions. The techniques in microfabrication, transfer printing and 3D shape definition are scalable to larger sizes and smaller, denser arrays of sensors. To increase the resolution and numbers of sensors, it may be necessary to incorporate transistors into the device to allow multiplexed addressing. Remaining challenges for use as a chronic implant include means for power supply, control/communication and encapsulation. These approaches present a promising opportunity to design and implement high-definition implantable devices for diagnostics and therapy of lethal heart diseases. Fabrication of 3D-MIMs The process, detailed in Supplementary Methods , starts with standard planar processing of inorganic semiconductor materials (Si, InGaN or AlInGaP) followed by transfer printing onto substrates coated either with a bilayer of polyimide (PI) on poly(methyl methacrylate) (PMMA) or poly(ethylene terephthalate) (PET) on poly(dimethylsiloxane) (PDMS) [15] , [27] , [28] , [29] , [30] . Dissolution of the PMMA or delamination from the PDMS allows release of the devices. Metal layers (Cr/Au) are vacuum-deposited and patterned to form interconnects, resistors and electrodes. Application and patterning of a polymer encapsulation layer (PI or a photosensitive epoxy, SU8) on top of the devices completes their fabrication. Transfer printing delivers the resulting structures to a thin film of a low-modulus silicone elastomer (Ecoflex, Smooth-on). A flexible conductive cable (Elform) bonded to contact pads at the periphery provides an interface to external hardware. A lamination process attaches the devices to a desired 3D-printed model of the heart, with the sensors in direct contact with the surface. Casting and curing another layer of the same type of elastomer defines the overall 3D geometry of the system ( Supplemental Fig. 16 ). In some cases, elastomer straps enhanced the manoeuvrability for use in Langendorff-perfused heart experiments ( Supplementary Fig. 14 ). Additional openings in the membrane can be included to prevent fluid build-up associated with flow in the supporting bath. Removal from the model allows electrodeposition of IrOx on to yield pristine surfaces for precision pH sensing. Mechanical analysis Numerical analysis by 3D FEM: The 3D FEM is used to study the pressure between the 3D-MIM and the heart for a wide range of device parameters and the expansion of the heart. The 3D geometric model of the heart is reconstructed from the data obtained with optical segmentation. The geometric model is imported into the pre-processor in the ABAQUS finite element program [31] . The heart and the 3D-MIM are modelled by the four-node, linear tetrahedron solid element C3D4 and the four-node quadrilateral membrane element M3D4 in ABAQUS, respectively. The total number of elements exceeds 60,000, and mesh refinement ensures the accuracy of the numerical results. For the prescribed expansion of the heart, FEM gives the pressure distribution at the interface between the 3D-MIM and the heart. The average pressure is then obtained over the contact area between the 3D-MIM and the heart, that is, the ventricles of the heart as in the experiment, as shown in Fig. 2a . Analytical calculations: The part of the heart that is covered by the 3D-MIM ( Fig. 2a ) is approximately a partial axisymmetric ellipsoid with the lengths a and b of semi-principal axes, as shown in Supplementary Fig. 1 . The 3D-MIM on the heart surface is modelled as a membrane, which deforms from Z 2 / a 2 + R 2 / b 2 =1 when being fabricated on the model to z 2 /((1+ ε ) 2 a 2 )+ r 2 /((1+ ε ) 2 b 2 )=1 due to the linear expansion ε of the heart, where ( Z , R ) and ( z , r )=((1+ ε ) Z , (1+ ε ) R ) are axial and radial coordinates of the 3D-MIM without and with expansion in the axisymmatric coordinates, respectively. The plane stress state of the 3D-MIM with biaxial linear strain gives the biaxial stress as E ε/(1− v ), where E and ν are the Young’s modulus and the Poisson’s ratio of the 3D-MIM, respectively. The membrane force, accounting for the change of length due to linear expansion, is where t is the thickness of the 3D-MIM. For a planar curve r = r ( z ), the principal curvature along the meridional direction is −(d r 2 /d z 2 )/(1+(d r /d z ) 2 ) 3/2 at any point ( z, r ) on the surface. The other principal curvature along the circumferential direction is given by . For z =(1+ ε ) Z and r =(1+ ε ) R , the two principal curvatures are given by The pressure on the heart is obtained in terms of the membrane tension and curvatures as in ref. 32 . Its average over the part of Z 0 ≤ Z ≤ a ( Supplementary Fig. 1a ) of the ellipsoid surface that is in contact with the heart is given by This gives Equation (1) in the main text, and For a =15 mm, b =10 mm and X 0 =−5.5 mm, which best fit the geometric model of the heart, the average pressure in Equation (1) agrees well with the 3D FEM results, as shown in Fig. 2b . The analysis above does not account for the effect of electronic devices on the pressure between the 3D-MIM and heart. Such an effect can be estimated from Equation (1) by replacing the tensile stiffness Et of the 3D-MIM with the effective tensile stiffness of the 3D-MIM with the electronic devices. The inset in Supplementary Fig. 1b shows an electronic device on a sheet of the membrane material (62.8 × 24.3 × 0.15 mm 3 ), consisting of the interconnects and electrodes. All of the interconnects consist of the Au: 120 nm/Cr: 2 nm composite layer sandwiched by 1.2-μm-thick P) layers on each side. The cross section of the electrodes is similar to that of interconnects but without the top 1.2-μm-thick PI layer to expose Au. The sheet is modelled by the eight-node solid element C3D8R, and interconnects and electrodes are modelled by the four-node shell element S4R in ABAQUS, respectively. FEM gives its tensile stiffness to be ~1.5 times that without the electronic devices, as shown in Supplementary Fig. 1b . Animal experiments Experiments were conducted in accordance with the ethical guidelines of the National Institutes of Health and with the approval of the Institutional Animal Care and Use Committee of Washington University in St Louis. Briefly, the heart is removed via a thoracotomy and a cannula is placed in the aorta to allow retrograde perfusion of oxygenated Tyrode’s solution. The perfusion mimics the electrolyte balance within the animal and provides an energy substrate for the heart to continue to function normally from an electrical perspective. The heart is submerged in a perfusion chamber maintained at 37 °C with a pH in the range of 7.35–7.45, controlled by oxygen flow. The optical signals of transmembrane potential ( V m ) and calcium transients (CaT) rely on the collection of fluorescent signals from a potentiometric dye (di-4 ANEPPS or RH-237) or calcium indicator (Rhod-2) added to the perfusate with a CMOS camera; when needed to avoid motion artifacts an excitation–contraction uncoupler (Blebbistatin) is also added to the perfusate. Supplementary Fig. 15 illustrates representative experimental settings. Data acquisition and processing Electrophysiology . The electrical signals are recorded from the Au electrodes on the 3D-MIMs with a 240-channel unipolar EG acquisition system (Astrocard, Boston) and a custom-built interface. Both the optical and electrical signals are collected at a sampling frequency of 1 kHz, aligned with a trigger TTL pulse and post-processed separately in custom MATLAB software. Post-processing: the electrical signals acquired from the 3D-MIMs are first filtered with a 60-Hz notch filter internal to the acquisition software, then the electrophysiological parameter of interest activation time is calculated ( Fig. 3c ) and aligned to the spatial coordinates of the electrodes based on the optical background file. The optical signals are binned, filtered and normalized as previously described [33] . A spatial 3 × 3 binning filter is applied, as well as a 100-Hz low-pass digital filter, and the amplitude of the fractional fluorescence is normalized to between 0 and 1 for each pixel’s temporal sequence. The electrophysiological parameters are calculated for the complete field of view. To create the spatial maps, the activation times are interpolated using MATLAB’s internal function for cubic interpolation of scattered data. The optical map is also sampled at the coordinates of the electrodes and the same interpolation method is applied to compare the full-resolution optical pattern with the sampled optical map and the electrical map. pH data pH data were acquired using measurement of open circuit potential of each sensor reference to an Ag/AgCl electrode, using Gamry Reference 600 potentiostat. A custom-made relay system was used for multiplexing. Temperature and strain Data for temperature and strain sensors are acquired with measurements of resistance of each sensor using a custom-built system based on National Instruments PXI-6289 board. The resistance of each of the 16 sensors is recorded simultaneously with a 160-μA probe current, a 16-bit A/D converter and a 15-ms sampling period at each sensor. How to cite this article: Xu, L. et al . 3D multifunctional integumentary membranes for spatiotemporal cardiac measurements and stimulation across the entire epicardium. Nat. Commun. 5:3329 doi: 10.1038/ncomms4329 (2014).